Assembly of a π–π stack of ligands in the binding site of an acetylcholine-binding protein Acetylcholine-binding protein is a water-soluble homologue of the extracellular ligand-binding domain of cys-loop receptors. It is used as a structurally accessible prototype for studying ligand binding to these pharmaceutically important pentameric ion channels, in particular to nicotinic acetylcholine receptors, due to conserved binding site residues present at the interface between two subunits. Here we report that an aromatic conjugated small molecule binds acetylcholine-binding protein in an ordered π–π stack of three identical molecules per binding site, two parallel and one antiparallel. Acetylcholine-binding protein stabilizes the assembly of the stack by aromatic contacts. Thanks to the plasticity of its ligand-binding site, acetylcholine-binding protein can accommodate the formation of aromatic stacks of different size by simple loop repositioning and minimal adjustment of the interactions. This type of supramolecular binding provides a novel paradigm in drug design. Screening compound libraries for biologically active molecules results in hit structures considered to be interesting starting points for drug design. Although it is often assumed that a single small drug molecule interacts with one protein-binding site, compounds binding to target proteins with higher stoichiometry can be found during library screening [1] . Here, we show an unexpected ligand interaction where three identical molecules interact within a single binding site. The binding of preorganized and/or in situ -organizing small binder molecules was shown to happen on the surface of proteins but examples of supramolecular assembly happening at the canonical-binding site of a target are still rare [2] , [3] . Recently two molecules of the IRE1 inhibitor quercetin were found binding at the dimer interface of the target and proved to induce its dimerization [4] (PDB: 3LJ0). An example of ligand supramolecular assembly was described also for a flavine-binding enzyme in complex with the cofactors FMN and NADH at the surface of the protein [5] (PDB: 2VZH, 2VZJ). Cys-loop receptors are important ligand-gated ion channels in the central and peripheral nervous systems [6] , [7] , [8] , [9] , [10] . Members include the nicotinic acetylcholine receptors (nAChR), GABA A receptors, 5HT 3 serotonin and glycine receptors, and all important pharmacological targets for various diseases and conditions [10] . nAChRs are targets for the endogenous neurotransmitter acetylcholine and for a series of compounds aimed at the treatment of cognitive decline in Alzheimer’s disease, certain forms of epilepsy [11] or nicotine addiction [12] . In the homo- or heteropentameric ion channels of the cys-loop receptor family, an extracellular ligand-binding site, is located at the interface between a ‘principal’ and a ‘complementary’ subunit, each of which contributes three loops (A–C and D–F, respectively) to the binding [6] , [7] , [8] , [13] . Agonist binding triggers conformational changes in cys-loop receptors and leads to opening of the channel and a flux of ions through the channel pore [14] . Ligand-binding sites in cys-loop receptors are highly plastic, allowing binding of various molecules ranging from small neurotransmitters all the way to large peptide neurotoxins, such as conotoxins and snake toxin [6] , [7] , [8] , [9] , [10] . Flexibility for different-sized ligands is generated by the positioning of loop C that contributes two conserved tyrosines and a vicinal disulphide bridge to the ligand-binding site. Most high-resolution structural information on cys-loop receptor–ligand interactions is available from a molluscan acetylcholine-binding protein (AChBP) [15] , [16] , [17] , [18] . AChBP structurally resembles the ligand-binding domains of cys-loop receptors, but lacks a transmembrane domain [16] . Their ligand-binding site resembles the α7 subtype of the nAChRs most (20–24% sequence identity) and their high-resolution crystal structures [16] , [17] , [18] , [19] , [20] , [21] , [22] , [23] reveal a structural fold closely related to cys-loop receptors as well as to their bacterial homologs [24] , [25] , [26] , [27] , [28] , [29] . Here we show that AChBP binds an ordered aromatic π–π stack of three identical ligands. The high-resolution X-ray crystal structure of this molecule in complex with Aplysia californica (Ac)-AChBP reveals a new example of protein–ligand interaction controlled by supramolecular ligand assembly. The nature of the binding mode, the analysis of protein residues contributing to the stabilization of the stack and the kinetics of the binding events are described. Finally, we identify acridine orange (AO) as a ligand with similar binding that could potentially be used as competitive inhibitor for α7 nAChR. 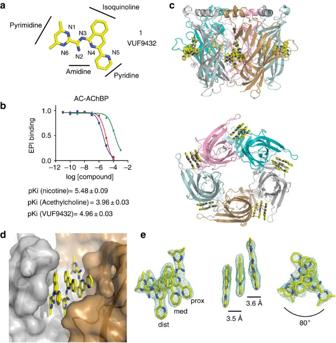Figure 1: VUF9432 binds as a triple stack to Ac-AChBP. (a) Chemical structure of VUF9432 (carbon atoms in yellow, nitrogen atoms in blue). (b) Displacement of radio-labelled epibatidine (EPI) by VUF9432 (red curves), nicotine (blue curves) and acetylcholine (green curves) on Ac-AChBP (purified proteins). Data are the mean±s.e.m. of three experiments and are reported below the panel. (c) Side and bottom side view of Ac-AChBP-VUF9432 complex structure, showing VUF9432 molecules (yellow sticks) in the five binding sites. (d) Protomer–protomer interfaces (surface representation) of Ac-AChBP-VUF9432 complex. Principal side is depicted in silver and complementary side in sand colours. Ligand-binding site are shown in transparency. (e) Electron density map displaying VUF9432 molecules in the ligand-binding site formed by subunit A and B (experimental density contoured at 1 σ), different orientation of the stacking molecules are shown together with the nomenclature used to distinguish the three molecules in the text. Intermolecular distances and angles are depicted as lines between the planes. dist, distal; med, medial; prox, proximal. Identification of VUF9432 A fragment [30] , [31] screening assay using online fluorescence enhancement led to the identification of fragments 2 – 6 ( Table 1 ) as hits for AChBP (refs. 32 , 33 ). In a subsequent analogue screening, VUF9432 ( 1) , (IUPAC name: 4,6-dimethyl- N -(3-(pyridin-2-yl)isoquinoline-1-yl)-pyrimidine-2-carboximidamide) ( Fig. 1a ) was shown to have micromolar affinity for AChBP. VUF9432 was originally synthesized as a copper-dependent antimycoplasmal agent active against Mycoplasma gallisepticum proliferation and later identified in a screen as ligand for adenosine A 3 receptors [34] . Table 1 Chemical formula, numbering and IUPAC name of the fragments. Full size table Figure 1: VUF9432 binds as a triple stack to Ac-AChBP. ( a ) Chemical structure of VUF9432 (carbon atoms in yellow, nitrogen atoms in blue). ( b ) Displacement of radio-labelled epibatidine (EPI) by VUF9432 (red curves), nicotine (blue curves) and acetylcholine (green curves) on Ac-AChBP (purified proteins). Data are the mean±s.e.m. of three experiments and are reported below the panel. ( c ) Side and bottom side view of Ac-AChBP-VUF9432 complex structure, showing VUF9432 molecules (yellow sticks) in the five binding sites. ( d ) Protomer–protomer interfaces (surface representation) of Ac-AChBP-VUF9432 complex. Principal side is depicted in silver and complementary side in sand colours. Ligand-binding site are shown in transparency. ( e ) Electron density map displaying VUF9432 molecules in the ligand-binding site formed by subunit A and B (experimental density contoured at 1 σ), different orientation of the stacking molecules are shown together with the nomenclature used to distinguish the three molecules in the text. Intermolecular distances and angles are depicted as lines between the planes. dist, distal; med, medial; prox, proximal. Full size image Binding affinities of VUF9432 for Ac-AChBP and α7 nAChR were measured in a radioligand displacement assay with [ 3 H] epibatidine and [ 3 H] methyllycaconitine (MLA) as displaceable ligands for AChBPs ( Fig. 1b ) and α7 nAChR ( Supplementary Fig. S1 ), respectively. VUF9432 behaves as competitive binder for AChBP, showing a pKi value of 4.96±0.03 for Ac-AChBP. The compound also displays some binding to α7 nAChR (pKi around five) but the radioligand is not fully displaced at the highest concentration tested, possibly due to low solubility of the compound under the assay conditions. In contrast to typical nAChR targeting molecules, VUF9432 lacks the canonical cation center involved in cation-π interactions with aromatic residues in the binding site [13] , [14] . The binding mode, interaction of VUF9432 to Ac-AChBP, was investigated by cocrystallization trials and X-ray analysis. VUF9432 binds AChBP in a triple stacked configuration The 2.4-Å crystal structure of the complex between Ac-AChBP and VUF9432 revealed the unexpected presence of three VUF9432 molecules in four out of the five ligand-binding sites in the pentamer (the fifth site is discussed separately below) ( Fig. 1c ). Careful refinement of the protein and the asymmetric shape of the VUF9432 molecule allowed the unambiguous fitting into the electron densities ( Fig. 1e and Supplementary Fig. 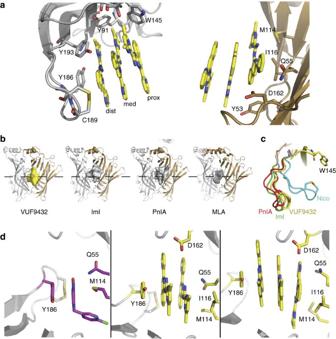Figure 2: Details of VUF9432 binding to Ac-AChBP. (a) Ball-and-stick representation showing Ac-AChBP residues on principal and complementary subunits interacting with VUF9432 (colours as in Fig. 1). The triple stack is held up like a row of books by Y186, Q55 and M114. Edge interactions with aromatic residues, D162 and the vicinal disulphide are indicated. (b) Protomer–protomer interfaces of VUF9432-Ac-AChBP structure illustrating how VUF9432 (surface, yellow) is occupying a lower part of the ligand-binding site if compared with the toxin IMI (surface, grey), PnIA (surface, grey) and MLA (surface, grey). (c) Comparison of C-loop opening in AChBP- nicotine (cyan), AChBP-PnIA (red), AChBP-IMI (green) and AChBP-VUF9432 (yellow) complex. Position assumed by the C-loop after VUF9432 binding resembles that in conotoxins. (d) Comparison of binding modes of Imidacloprid (magenta) and VUF9432 (yellow) to AChBP showing the two ligands establishing similar interactions with the ligand-binding site. Repositioning of the C-loop provides the space for either one, two or three flat aromatic moieties. S2 ), resulting in a refined structure with R =21%/ R free =25% and excellent stereochemistry ( Table 2 ). Table 2 Data collection and refinement statistics. Full size table Within each ligand-binding site, the three conjugated molecules of VUF9432 stack on each other ( Fig. 1e ) in a flat planar configuration. The three molecules are organized in a columnar stack, with an off-centred parallel displaced geometry. The distal molecule of VUF9432, closest to the C-loop and the medial one ( Fig. 1e ) are identically oriented with the pyrimidine rings pointing towards the inner part of the ligand-binding site, whereas the proximal molecule is twofold rotated relative to the other VUF9432 molecules. The distance between the medial molecule and the proximal and distal ones are 3.5 and 3.6 Å, respectively, consistent with previously measured π–π stacking distances between aromatic molecules [35] . The angle between the planes is at most 3.8±0.8° and 6.2±2.1°, due to slight tilting of the medial and proximal molecules towards the distal one, respectively, confirming the almost perfectly parallel displaced orientation ( Fig. 1e ). The proximal and distal copies of the molecule occupy slightly variable tilt angles within these planes, and hence have somewhat higher average B factors (58.4±10.23, 60.28±10.16 and 74.45±11.8 Å 2 for the medial, proximal and distal copy of VUF9432, respectively). Nevertheless it is clear that all three sites are fully occupied and the excellent quality of the electron density of the C-loop indicates full occupancy of these ligands. The stack of aromatic VUF9432 molecules is held in place like a pile of books, at one end by the stacking of well-conserved principal face residue Y186 ( Fig. 2a ), which has an off-centred displaced parallel π–π interaction with the distal molecule, tilted at 12.3±2.4°. At the other end the stack is positioned through van der Waals interactions with complementary side residues Q55 and M114. The side chain of I116 is positioned towards the stack, but does not interact with the proximal molecule. Figure 2: Details of VUF9432 binding to Ac-AChBP. ( a ) Ball-and-stick representation showing Ac-AChBP residues on principal and complementary subunits interacting with VUF9432 (colours as in Fig. 1). The triple stack is held up like a row of books by Y186, Q55 and M114. Edge interactions with aromatic residues, D162 and the vicinal disulphide are indicated. ( b ) Protomer–protomer interfaces of VUF9432-Ac-AChBP structure illustrating how VUF9432 (surface, yellow) is occupying a lower part of the ligand-binding site if compared with the toxin IMI (surface, grey), PnIA (surface, grey) and MLA (surface, grey). ( c ) Comparison of C-loop opening in AChBP- nicotine (cyan), AChBP-PnIA (red), AChBP-IMI (green) and AChBP-VUF9432 (yellow) complex. Position assumed by the C-loop after VUF9432 binding resembles that in conotoxins. ( d ) Comparison of binding modes of Imidacloprid (magenta) and VUF9432 (yellow) to AChBP showing the two ligands establishing similar interactions with the ligand-binding site. Repositioning of the C-loop provides the space for either one, two or three flat aromatic moieties. Full size image Aromatic groups on the principal (Y91, W145, Y193) and complementary faces (Y53) stabilize the sides of the stack of ligands via edge-to-face interactions, establishing T-shaped aromatic contacts with the molecules ( Fig. 2a ). Finally, the F-loop D162 and the vicinal disulphide in the C-loop also interact with the sides of the stacked VUF9432 molecules. Taken together, the three stacked molecules of VUF9432 occupy a large volume and bury a substantial surface area in AChBP (959.9±4.8 Å 2 ) comparable with the area buried by conotoxins IMI [20] (PDB:2C9T) and PnIA [19] (PDB:2BR8) (1164 Å 2 and 1468 Å 2 , respectively). However, the position of VUF9432 in the binding site is different, as can be seen in Fig. 2b . The space occupied by the conotoxins is above the midline of the pentamer, away from the transmembrane domain in the cys-loop receptors, whereas the VUF9432 molecules are placed lower, close to the membrane, not far from the binding site for MLA (ref. 36 ). However, MLA (PDB:2BYR) is in a different site closer to the five-fold axis than VUF9432, which uses a lower, more external cavity ( Fig. 2b ). It does not address the so-called ‘lobeline pocket’ and Y91 is in the g-conformation, interacting with S144 [37] . The combination of this novel position and slightly smaller buried surface area result in a C-loop position that is similar to that for the conotoxins, in its most open state ( Supplementary Fig. S3 ). In one of the five ligand-binding sites only two molecules of VUF9432 are bound, positioned in parallel manner, similarly to the medial and the distal copy in the other ligand-binding sites ( Fig. 3a ). This state is most likely stabilized by crystal contacts ( Fig. 3f ). Although the double stack is tilted 15°relative to the triple stack in the other binding sites ( Fig. 3c ), the direct contacts are retained. Thus, the stack is upheld by Y186 at one end and M114 and Q55 at the other end with similar side interactions ( Fig. 3d ). The major difference for this binding site is caused by the loop C position, which in this case is in an intermediate open state, similar to that found for ligands such as tubocurarine [38] (PDB:2XYT) and α-cobratoxin [39] (PDB:1YI5) ( Fig. 3e ). 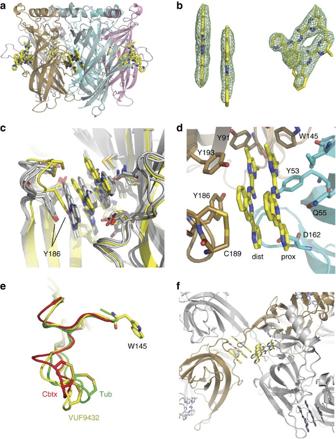Figure 3: AChBP can accommodate a double stack of VUF9432. (a) Side view of Ac-AChBP-VUF9432 complex structure, showing two VUF9432 molecules (yellow sticks) in the binding site formed by subunit B (sand) and C (cyan). (b) Electron density map displaying VUF9432 molecules in the ligand-binding site formed by subunit B and C (experimental density contoured at 1 σ). (c) Superposition of the four ligand binds site binding triple stacks of VUF9432 (grey cartoon and sticks) and the one binding the double stack of molecule (yellow cartoon and sticks), showing the movement of the Y186 to accommodate the third molecule of the stack. (d) Ball-and-stick representation showing AChBP residues on principal and complementary subunits interacting with the double stack of VUF9432 (colours as ina). (e) Comparison of C-loop opening in AChBP-tubocurarine (Tub, green), AChBP-α-cobratoxin (Cbtx, red), AChBP-VUF9432 (the shown C-loop is the one of the ligand-binding site containing two copies of the stack, yellow) complex. Position assumed by the C-loop after VUF9432 binding resembles that in cobratoxin. (f) Interaction of an AChBP-VUF9432 molecule with the symmetry-related molecule that form intermolecular contacts. The open C-loop of subunit B contacts the F-loop of a symmetry-related molecules. The bound VUF9432 molecules are shown in ball and sticks. Figure 3: AChBP can accommodate a double stack of VUF9432. ( a ) Side view of Ac-AChBP-VUF9432 complex structure, showing two VUF9432 molecules (yellow sticks) in the binding site formed by subunit B (sand) and C (cyan). ( b ) Electron density map displaying VUF9432 molecules in the ligand-binding site formed by subunit B and C (experimental density contoured at 1 σ). ( c ) Superposition of the four ligand binds site binding triple stacks of VUF9432 (grey cartoon and sticks) and the one binding the double stack of molecule (yellow cartoon and sticks), showing the movement of the Y186 to accommodate the third molecule of the stack. ( d ) Ball-and-stick representation showing AChBP residues on principal and complementary subunits interacting with the double stack of VUF9432 (colours as in a ). ( e ) Comparison of C-loop opening in AChBP-tubocurarine (Tub, green), AChBP-α-cobratoxin (Cbtx, red), AChBP-VUF9432 (the shown C-loop is the one of the ligand-binding site containing two copies of the stack, yellow) complex. Position assumed by the C-loop after VUF9432 binding resembles that in cobratoxin. ( f ) Interaction of an AChBP-VUF9432 molecule with the symmetry-related molecule that form intermolecular contacts. The open C-loop of subunit B contacts the F-loop of a symmetry-related molecules. The bound VUF9432 molecules are shown in ball and sticks. Full size image Interestingly, these contacts resemble those described for the pentameric ring of imidacloprid [40] , [41] . In that case, the flat aromatic imidazolinic part of the molecule is held in place by face to face stacking with Y186 and upheld by van der Waals contacts with M114. A H-bond connects the Q55 to an oxygen of the nitro group of imidacloprid ( Fig. 2d ), now held in place by a maximally closed C-loop. Here, we show that the binding site of AChBP provides space for either one, as in imidacloprid, two or three flat aromatic moieties as seen here for VUF9432, all with similar contacts. This remarkable plasticity is organized primarily by repositioning of the C-loop ( Fig. 2d ). Ligand stacking promoted by aromaticity and planarity To exclude that the unusual configuration of these ligands is a crystallographic artifact, we analysed the binding in several ways. First we confirmed the VUF9432 binding to the ligand-binding site, by mutating interacting amino acids. Mutation of either Y186 or Y193 to alanine resulted in the loss of affinity for VUF9432 ( Supplementary Fig. S4 ), confirming, also in solution, the binding to the canonical pocket. We then tested the stoichiometry of VUF9432 binding to Ac-AChBP in solution, using equilibrium titration. Binding was analysed by the change in the fluorescence emission of W145 of AChBP, which correlates with the binding of agonists or antagonists [42] . Titration of nicotine binding at high protein concentrations showed that the fluorescence quenching reaches a plateau at the stoichiometric ratio ligand/AChBP close to one nicotine molecule bound per protomer ( Fig. 4b ). In contrast the titration profile of VUF9432 binding does not saturate until a stoichiometry of three ligands per protomer is reached ( Fig. 4d ), confirming the crystallographic data. 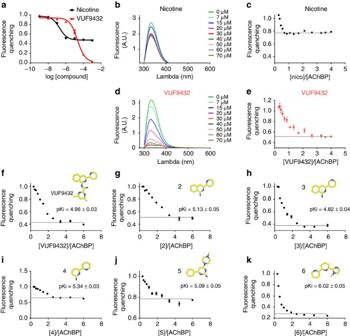Figure 4: Aromaticity and planarity determine multiple ligand binding to AChBP. (a) Comparison of affinity of Ac-AChBP for VUF9432 (red curve) and nicotine (black curve) measured with tryptophan fluorescence quenching. Titration of binding sites for nicotine (b,c) and VUF9432 (d,e) on Ac-AChBP by fluorescence quenching. Ac-AChBP at 20 μM binding sites was titrated with incremental quantities of ligand. Fluorescence excitation was at 280 nm. Full emission spectra were recorded and maxima were measured over the range 335–345 nm (b,d) and plotted versus the nicotine/AChBP (c, black dots) or VUF9432/AChBP (e, red dots) stoichiometric ratio. A straight line was fit through the plateau points (grey line) as described in the methods section. (f–k) Titration of binding sites for the VUF9432 and analogues on Ac-AChBP by fluorescence quenching. Affinity for AChBP (mean±s.e.m. measured with radiodisplacement assay) and structure of the ligands (colours as in figure 1) are indicated. AChBP at 20 μM was titrated with incremental quantities of ligands as described above (fluorescence maxima plotted as inc). Figure 4: Aromaticity and planarity determine multiple ligand binding to AChBP. ( a ) Comparison of affinity of Ac-AChBP for VUF9432 (red curve) and nicotine (black curve) measured with tryptophan fluorescence quenching. Titration of binding sites for nicotine ( b , c ) and VUF9432 ( d , e ) on Ac-AChBP by fluorescence quenching. Ac-AChBP at 20 μM binding sites was titrated with incremental quantities of ligand. Fluorescence excitation was at 280 nm. Full emission spectra were recorded and maxima were measured over the range 335–345 nm ( b , d ) and plotted versus the nicotine/AChBP ( c , black dots) or VUF9432/AChBP ( e , red dots) stoichiometric ratio. A straight line was fit through the plateau points (grey line) as described in the methods section. ( f – k ) Titration of binding sites for the VUF9432 and analogues on Ac-AChBP by fluorescence quenching. Affinity for AChBP (mean±s.e.m. measured with radiodisplacement assay) and structure of the ligands (colours as in figure 1) are indicated. AChBP at 20 μM was titrated with incremental quantities of ligands as described above (fluorescence maxima plotted as in c ). Full size image We wondered what properties of VUF9432 are necessary for the supramolecular binding. Conformational analysis in the gas phase ( Supplementary Fig. S5a ) shows that VUF9432 can adopt a series of relatively planar conformations, with minimal rotational freedom of the pyridine ring and of the amidine bond. In the structure a conformation is selected where the pyridine, isoquinoline and pyrimidine rings are coplanar stabilized by a hydrogen bond between the amidine N2 and the isoquinolinic N4. We then analysed the original fragment hits for their ligand-binding stoichiometries using fluorescence quenching. Affinity of these fragments for Ac-AChBP was relatively weak ( Supplementary Fig. 6 , numbers presented as mean pKi in Fig. 4f–k ), which meant that we could only use a relative small excess of Ac-AChBP in these experiments. Nevertheless, we could clearly observe that several fragments retain the ability to bind in a three-to-one ratio. Derivatives,VUF6141 ( 2) and VUF5954 ( 3) ( Fig. 4g ), that lack the pyrimidine ring show similar affinity to Ac-AChBP compared with VUF9432, in line with the lack of interaction with Ac-AChBP for this moiety. In computational analysis, both compounds are able to adopt a planar configuration ( Supplementary Fig. S5b ,c), especially compound 2 , where the planar configuration is the most stable, thanks to the N in position 6 of the pyridine, that prevents clashing between the hydrogen atoms of the isoquinolinic and the pyridine rings ( Supplementary Fig. S5b ,c). Equilibrium fluorescence titration clearly indicates that Ac-AChBP can bind multiple copies of ligand 2 and 3 per binding site ( Fig. 4g ). Interestingly, supramolecular binding was also seen for the bi-pyrimidinic compound VUF11370 ( 4) ( Fig. 4i ) showing that different aromatic planar molecules can self-assemble in Ac-AChBP. As seen for 2 , compound 4 prefers the planar conformation ( Supplementary Fig. S5d ). In compound VUF10460 ( 5 ), a piperazine moiety is present. As seen for nicotine ( Fig. 4c ) and many other canonical AChBP ligands [42] , this compound induces less fluorescence quenching after binding to AChBP. Equilibrium fluorescence titration indicates the stoichiometry is changed to 1:1, although the affinity for the receptor was maintained ( Fig. 4j ). This molecule is not fully aromatic resulting in non-planarity of the piperazine moiety ( Supplementary Fig. S5e ), which most likely prevents the stacking observed in compounds 1 – 4 . Moreover, the compound is slightly basic, which could allow a cation-π interaction and an alternative binding mode. The presence of an imidazolinic moiety like in compound VUF14476 ( 6 ) could result in a loss of the binding of multiple copies ( Fig. 4k ). In compound 6 , the methyl group attached to the imidazole ring is located at the centre of the molecule ( Supplementary Fig. S5f ), possibly preventing the formation of stacked molecules. Although there are two methyl groups present on the pyrimidine ring of VUF9432, these are at the edge of the molecule. The slight displacement of the molecules in the stacks may just be enough to ensure the absence of clashes between the hydrogen atoms of the methyl present on the distal and the medial molecules, when located at the edge of the molecule. Even assembling in a similar displaced configuration, the clashes between the hydrogen atoms of the methyl group of 6 could probably not be avoided, explaining the one to one stoichiometry to AChBP. Binding of VUF9432 molecules occurs in steps An interesting question is whether the three molecules bind as a ‘package’ or whether they bind sequentially. For this we first analysed the shape of the binding curves of the three molecules in VUF9432 and derivatives 2 – 4 ( Fig. 4a ), some of which may be non-linear. This non-linearity could reflect differences in affinities for the three VUF9432 sites, resulting in differently shaped binding curves. Alternatively, the effect of binding of the three individual molecules could have differential effects on the tryptophan quenching. One could even imagine that a stack of more than one ligand will receive increased levels of resonance energy transferred from remote aromatic residues, otherwise unaffected by the binding of a single molecule. It will not be trivial to uncouple these possibilities, but it seems likely that the binding event is not a single-step transition of a single package of three ligands into the binding site. To analyse the binding process in more detail, we used stopped-flow kinetic studies to monitor this assembly process ( Fig. 5 ). Titration of nicotine shows simple association to Ac-AChBP ( Fig. 5a ) [42] that can be fitted with a one-step binding model ( Fig. 5d ). In contrast, the binding profile of VUF9432 cannot be fitted with a simple model ( Fig. 5b ). In practice a two-step fitting of the binding is sufficient to achieve acceptable residuals ( Fig. 5e ), confirming a more complex binding process. In contrast to the proposed binding of bungarotoxin [42] , where the second step is concentration independent and most likely due to a conformational adjustment, for VUF9432 the second step varies with concentration, indicating the stepwise binding of the ligands. 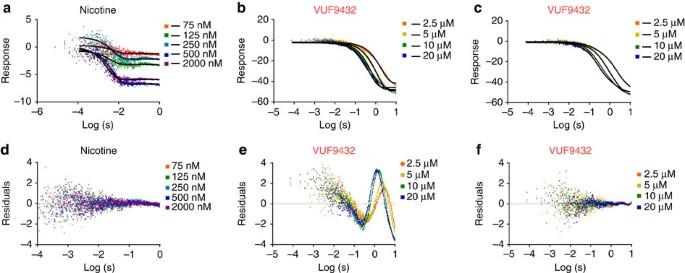Figure 5: Binding of VUF9432 is a multistep process. Kinetic studies of ligand association with AChBP. Stopped-flow traces of tryptophan fluorescence quenching on Ac-AChBP binding to nicotine (a) and VUF9432 (b,c). Upper panels show typical traces of observed fluorescence during and after stop page of flow at the indicated ligand concentrations. Paneldreports the residuals of the fitting for one-step nicotine binding to AChBP. Panelseandfreport the residuals of the fitting for one (e) or two steps binding (f) of VUF9432 to AChBP, respectively. Figure 5: Binding of VUF9432 is a multistep process. Kinetic studies of ligand association with AChBP. Stopped-flow traces of tryptophan fluorescence quenching on Ac-AChBP binding to nicotine ( a ) and VUF9432 ( b , c ). Upper panels show typical traces of observed fluorescence during and after stop page of flow at the indicated ligand concentrations. Panel d reports the residuals of the fitting for one-step nicotine binding to AChBP. Panels e and f report the residuals of the fitting for one ( e ) or two steps binding ( f ) of VUF9432 to AChBP, respectively. Full size image Multiple binding of a fluorescent aromatic molecule to AChBP We wondered whether different molecules could bind in this manner and searched for planar aromatic molecules. AO [43] , [44] , [45] is a fluorescent planar aromatic molecule with increased solubility compared with VUF9432. We found that AO ( Fig. 6a ) binds the ligand-binding site of AChBP with micromolar affinity (pKi=5.8, Fig. 6b ). An analogue of AO, N -methylacridinium, was shown to bind in the active site of the enzyme acetylcholinesterase, which also displays affinity for acetylcholine [46] . When AO binding to Ac-AChBP was tested using tryptophan fluorescence quenching at high concentration, we observed that as for VUF9432 the binding has a stoichiometric ratio higher than one ( Fig. 6c ). In agreement with this, titration of Ac-AChBP into an AO solution, Ac-AChBP quenched AO fluorescence at a stoichiometric ratio of 0.3 ( Fig. 6d , black dots). This quenching of AO by Ac-AChBP is inhibited in the presence of an excess of nicotine, confirming that AO is binding competitively to the binding pocket of Ac-AChBP ( Fig. 6d , grey dots). 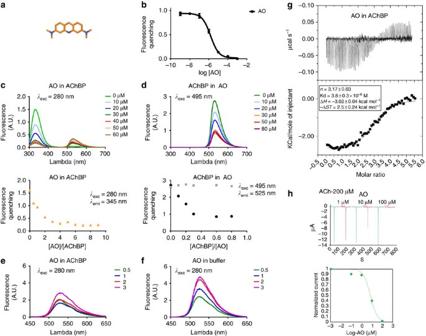Figure 6: AO orange mimics the triple stacking ligand. (a) Chemical structure of AO (carbon in orange, nitrogen in blue) (b) Affinity of Ac-AChBP for AO measured with fluorescence quenching (as described in Figure4). (c) Titration of binding sites for AO on Ac-AChBP by tryptophan fluorescence quenching. Ac-AChBP at 20 μM was titrated with incremental quantities of AO. Fluorescence excitation was at 280 nm and full emission spectra were collected between 300 and 700 nm, and emission maxima were measured over the range 335–345 nm and plotted versus the AO/AChBP stoichiometric ratio. (d) Titration of binding sites for AO on Ac-AChBP by AO fluorescence quenching. AO at 100 μM was titrated with incremental quantities of AChBP in presence (grey dots) or in absence of 1 mM nicotine (black dots). Fluorescence excitation was at 495 nm and full emission spectra were collected between 300 and 700 nm: emission maxima were measured over the range 525–535 nm and plotted versus the AO-AChBP stoichiometric ratio. Comparison of the fluoresce emission of free AO (f) or AChBP-AO complex (e) at stoichiometric ratio AO-AChBP of 0.5 (green curve), 1 (blue curve), 2 (red curve) and 3 (purple curve). (g) Calorimetric data of AO binding to AChBP. Top panel shows the raw heat measured over a series of AO injections (500 μM). Each heat signal is integrated and shown as data point in the bottom panel. Data points were fitted to a model describing a single set of binding sites and best-fit parameters for AO binding were calculated using least-squares fitting. (h) Acridine orange inhibits half of ACh-evoked currents at α7 nAChR receptors expressed in oocytes at concentrations around 10 μM and gives almost full inhibition of the current at 100 μM. Figure 6: AO orange mimics the triple stacking ligand. ( a ) Chemical structure of AO (carbon in orange, nitrogen in blue) ( b ) Affinity of Ac-AChBP for AO measured with fluorescence quenching (as described in Figure4). ( c ) Titration of binding sites for AO on Ac-AChBP by tryptophan fluorescence quenching. Ac-AChBP at 20 μM was titrated with incremental quantities of AO. Fluorescence excitation was at 280 nm and full emission spectra were collected between 300 and 700 nm, and emission maxima were measured over the range 335–345 nm and plotted versus the AO/AChBP stoichiometric ratio. ( d ) Titration of binding sites for AO on Ac-AChBP by AO fluorescence quenching. AO at 100 μM was titrated with incremental quantities of AChBP in presence (grey dots) or in absence of 1 mM nicotine (black dots). Fluorescence excitation was at 495 nm and full emission spectra were collected between 300 and 700 nm: emission maxima were measured over the range 525–535 nm and plotted versus the AO-AChBP stoichiometric ratio. Comparison of the fluoresce emission of free AO ( f ) or AChBP-AO complex ( e ) at stoichiometric ratio AO-AChBP of 0.5 (green curve), 1 (blue curve), 2 (red curve) and 3 (purple curve). ( g ) Calorimetric data of AO binding to AChBP. Top panel shows the raw heat measured over a series of AO injections (500 μM). Each heat signal is integrated and shown as data point in the bottom panel. Data points were fitted to a model describing a single set of binding sites and best-fit parameters for AO binding were calculated using least-squares fitting. ( h ) Acridine orange inhibits half of ACh-evoked currents at α7 nAChR receptors expressed in oocytes at concentrations around 10 μM and gives almost full inhibition of the current at 100 μM. Full size image The formation of the AO stack in Ac-AChBP should determine differences in the emission spectra of the molecules as seen for aromatic π–π stacking in organic aromatic cages [47] . The fluorescence spectra of AO in complex with Ac-AChBP and those free in solution were compared. Emission at 525nm (π–π* transition) [43] of the complexed acridine moiety is quenched in the presence of Ac-AChBP due to the interaction of AO with the aromatic environment. During the titration the intensity at 525 nm increases without further shifts ( Fig. 6f ), as expected [47] . AO is highly soluble allowing us to use isothermal titration calorimetry (ITC) to follow its binding to AChBP. Our data indicate that AO binds to Ac-AChBP with a stoichiometric ratio of 3–4, with a Kd of 1.86 μM and that the sequential binding is enthalpically favoured ( Fig. 6g ). Fitting of the experimental data to a model indicates the existence of three events of AO binding per ligand-binding domain of Ac-AChBP. This confirms that other planar molecules can bind to the Ac-AChBP ligand-binding site in a similar manner to VUF9432. Interestingly, when AO was tested in electrophysiology experiments on α7 nAChR-expressing oocytes, it behaved as competitive inhibitor with an IC50 of 7.3 μM, showing an affinity similar to the one measured for Ac-AChBP ( Fig. 6h ). Thus, ligands with the potential of supramolecular binding can be relevant for drug design on nAChRs. To our knowledge Ac-AChBP is the first example of a target protein binding a triple π–π stack of ligand molecules. In this paper, we prove that Ac-AChBP binds VUF9432 ( Figs 1 , 2 , 3 , 4 , 5 ), fragments 2 , 3 , 4 , and AO with stoichiometry higher than one ( Figs 4 and 6 ). All these compounds address the canonical-binding site of Ac-AChBP and behave as competitive binders ( Figs 1 , 4 and 6 ). Aromaticity and planarity of the molecule positively influence the super-stoichiometry ( Fig. 4 and Supplementary Fig. S5 ). VUF9432 is not very soluble and binds only weakly to α7 nAChR. When tested in electrophysiology experiments, we did not observe any effect of VUF9432 on α7 nAChR expressed in oocytes, probably due to the low solubility (data not shown). However, we identified AO as a molecule that binds AChBP with similar binding properties and stoichiometry. Interestingly, this highly soluble ligand has robust inhibitory properties on nAChR in oocytes, showing the potential for exploitation of these types of ligand binding. The crystal structure of VUF9432 in Ac-AChBP allows analysis of the supramolecular binding mode. The three molecules of VUF9432 stack in a parallel displaced orientation. The latter was reported to be one of the lowest energetic conformations that such a stack can acquire [35] . In addition several edge-to-face interactions are observed, contributing to the binding properties. The non-linearity of the binding curves of VUF9432, compound 2 – 4 and AO, the stopped-flow analysis of VUF9432 binding to Ac-AChBP and the ITC measurement of AO binding to Ac-AChBP suggest that likely the stacking of the molecules is happening in situ and not as preassembled stack ( Figs 4 , 5 , 6 ). However, we cannot exclude other scenarios. Stopped-flow fluorescence measurement of the binding of α-bungarotoxin to Ac-AChBP was shown to not be a one-step event [43] . This result was interpreted, suggesting multiple binding modes of the toxin to the binding site of Ac-AChBP. As postulated for the toxin also a stack of VUF9432 could just bind preassembled and have multiple binding modes. Conformational search performed in gas phase would suggests that this unusual stacking is not present for VUF9432 in solution and that the assembly in situ at the protein-binding site would be energetically more favoured. In particular, the dipole on VUF9432 would disfavour the parallel stacking that is observed for the distal and medial copies of the compound ( Figs 1 , 2 , 3 ). Hence, it is clear that interactions with Ac-AChBP could contribute to stabilize these configurations and that each VUF9432 molecule orients in the ligand-binding site according to the electrostatic environment of the protein rather than their individual local dipole moment. Entropic factors hamper the intentional creation of parallel π–π stacks of molecules. ‘Tweezer’ molecules have been used to stabilize columns of aromatic molecules [48] . Also, reconstitution of a discrete columnar stack of aromatic molecules has been achieved using box-shaped coordination cage [47] . Here, we show that a protein can enable the formation of a π–π stack of molecules. The stacking is stabilized by the contribution of the aromatic side chains of the ligand-binding site. Although π–π interactions are thought to be weak [35] , they have been recognized to have an important role in the folding and in the thermal stability of proteins and the binding to ligands. The binding site in Ac-AChBP is closely related to that of other cys-loop receptors, where specificity for different ligands is provided by amino-acid changes in the loops A–C and D–F. The remarkable plasticity of the ligand-binding site, allowing the binding of differently sized ligands in cys-loop receptors, is tuned by the positioning of the C-loop and has a pivotal role in dictating the dimension of the stack. Recently, Ac-AChBP was found to be capable of accommodating two molecules of acetylcholine it its binding sites, although relative occupancies are very different between the two molecules [49] (PDB: 2XZ5). Here, we show that the binding site offers a variety of binding possibilities, by simple repositioning of the C-loop ( Figs 2 and 3 ) to accommodate either one, two or three ligand molecules ( Fig. 2 ), with relatively little adjustment in the interactions. The binding site AChBP was recently shown to accommodate in situ Huisgen cycloaddiction ‘click’ reactions [50] . Thus, these binding sites can serve as a reaction vessel for chemical reactions. In combination with the ability to promote supramolecular self-assembly, this binding site provides a unique environment for novel chemistry, which can be further tuned by amino-acid variations of loops A–F, varying the properties of the binding pocket. Multiple binding in a specific manner within a ligand-binding site provides a novel paradigm for ligand binding. Aggregation of molecules and the presence of multiple independent binding sites have been discussed in the area of drug design previously [51] . However, the interdependent binding required to make a ligand stack is different. It provides specific opportunities as well as novel challenges. Clearly, it will become important to take the stacking possibility into account when analysing ligand binding. Stoichiometry analysis will be important, in particular when considering binding profiles that could potentially provide this type of stacking. Meanwhile, one can see this as a novel opportunity, providing previously unexplored avenues for drug design. Not necessarily trivial, as large flat molecules have obvious disadvantages in design strategies compared with three-dimensional fragments [51] , but definitely a new and unexplored opportunity, where a ligand induces different opening of a ligand-binding site while establishing the same interactions with the target protein. In addition, the growing literature on ‘tweezer’ molecules [48] and on biocatalytic induction of supramolecular order [52] may well prove helpful in exploring the possibilities of purposely designing stacks of ligands in proteins. Proteins Untagged wild-type (wt) and mutants Ac-AChBPs were purified from Sf21 insect cells as previously described [19] . The complementary DNAs for the Ac-AChBP mutants, Ac-AChBP Y186A and Ac-AChBP Y193A, were generated using Quik Change Mutagenesis following the manufacturer’s protocols. Mutant proteins were expressed from baculovirus in Sf21 cells. SHS5Y neuroblastoma cell membranes were used as source of α7 nAChR in radiodisplacement assays [15] . Conformational search A stochastic conformational search was performed using MOE (version 2011.10, Chemical Computing Group Montreal, Canada), using default settings. Crystallization The VUF9432-Ac-AChBP complex was formed by mixing the protein at 3.5 mg ml −1 with 1 mM VUF9432 and incubating on ice for 1 h. Cocrystals were grown using the vapour diffusion method in a solution consisting of 0.2 M Li 2 SO 4 and 0.8 M ammonium sulphate in MMT buffer (pH 8.0) at 19 °C. Crystals were cryoprotected in mother liquor supplemented with 20% glycerol and flash-frozen in liquid nitrogen. Structure solution and refinement Data were collected on beamline PX1 at the SLS (Switzerland), and processed using iMOSFLM/SCALA software [55] . The VUF9432-Ac-AChBP cocrystal was in space group P2 1 and diffracted to a resolution of 2.4 Å. The structure was solved by molecular replacement using PHASER [53] and the Ac-ACHBP-HEPES structure (2BR7) (ref. 19 ) as model. Iterative structure refinement was performed using REFMAC [54] from the CCP4 suite [56] or BUSTER [57] . Non-crystallographic symmetry restraints (NCSR) were maintained during refinement, using local NCS restraints as implemented in REFMAC or local structure similarity restraints in BUSTER. One TLS group per chain was used in refinement, and both the X-ray weight and B-factor restraint weight were optimized using a local version of the PDB_REDO script [58] . Ligands and water molecules were built in the final stages of refinement. Validation, performed using molprobity [59] and PDB_REDO, identified 0% of Ramachandran outliers and 2% of poor rotamers (overall score: 99th percentile). Distances, angles and buried surface areas were measured in Pymol (DeLano Scientific, LLC). Values and errors in text refer to the average over the four ligand-binding sites with three ligands bound. C-loop opening was calculated measuring the distance between Nε of W145 and Sγ of Cys 189. Tilting angles of aromatic planes was obtained by calculating the angle between the normal to the planes and averaged over four ligand-binding sites. Ligand radiodisplacement assays Competition binding assays were performed with Ac-AChBP (wt or mutants) in buffer (PBS, 20 mM Tris, pH 7.4/0.05% Tween) in a final assay volume of 100 μl in Optiplates (PerkinElmer Life Science, Inc., USA). Ligands were added at 10 −3 –10 −11 M. Radioligand, [ 3 H] epibatidine (PerkinElmer, specific activity ~56 Ci mmol −1 ), was added at 2.25 nM. The amount of protein was chosen such that we obtained a counting window in the displacement curve of <5% of the total amount of radioligand, generally 2–20 ng. Copper His-Tag PVT SPA beads (PerkinElmer) were added at 2 mg ml −1 final concentration. Plates were incubated at room temperature under continuous shaking, protected from light, for 1.5 h. SPA beads were allowed to settle for 3 h in the absence of light before counting. The label-bead complex was counted in a Wallac Trilux 1450 Microbeta (PerkinElmer). Binding assays with α-bungarotoxin-[ 125 I] (IBTX) were performed as above at 1.8 nM IBTX. Binding assays with the human α7 receptor were performed as above, but without the SPA beads, as a filtration assay. Human neuroblastoma cells (SH-SY5Y) expressing human α7 nAChRs (from Christian Fuhrer, Department of Neurochemistry, Brain Research Institute, Zurich) were cultured. The cells were washed three times, and pelleted aliquots were stored frozen at –80 °C. Before use the cells were resuspended in ice-cold buffer and sonicated. [ 3 H]MLA (American Radiolabeled Chemicals, Inc., specific activity ~100 Ci mmol −1 ) was used at a final concentration of 2 nM. Bound radioligand was collected on 0.3% polyethyleneimine-pretreated Unifilter-96 GF/C filters (PerkinElmer). Plates were washed with ice-cold 50 mM Tris buffer at pH 7.4. After drying the filters, scintillation fluid (MicroScint, PerkinElmer) was added and the radioactivity was counted as above. All radioligand binding data were evaluated by a non-linear, least-squares curve fitting procedure using GraphPad Prism (version 5, GraphPad Software, Inc., San Diego, CA). All data are represented as mean±s.e.m. from at least three independent experiments. Trp and AO fluorescence quenching Ac-AChBP, 1 μM in binding site, was equilibrated with dilution of the ligands 1 h before fluorescence measurement. Equilibrium fluorescence was monitored using a PheraStar fluorescence plate reader in the 96-well plates. Ac-AChBP was excited at 280 nm, and emission intensity was monitored at 340 nm with an emission slit of 8 nm. AO was excited at 495 nm and emission monitored at 525 nm with an emission slit of 10 nm. Data were normalized, and pKi values were calculated by fitting to a sigmoidal dose–response curve with GraphPad. To determine ligand stoichiometries, Ac-AChBP (20 μM in binding site) was titrated with increasing concentration of ligand until <8% quenching was apparent. A straight line was fit through the average of the plateau points. For AO titration by Ac-AChBP, AO (100 μM) was titrated with increasing concentration of protein. When indicated 1 mM nicotine was added to the assay to compete with AO. Full fluorescence spectra were recorded with a QuantaMaster 3 Fluorometer. Isothermal calorimetry ITC experiments were performed on a VP-ITC microcalorimeter (Microcal) at 25°as described [17] . Ac-AChBP used in these experiments was dialysed in PBS, and the AO was solubilized in the same buffer. For a typical experiment, the ligand at a concentration of 0.5 mM was titrated into 20 μM Ac-AChBP. Titration of ligand in buffer alone was performed to determine the change in enthalpy caused by the dilution of the ligand and subtracted as background from the actual ligand-binding experiment. Corrected data were analysed using software supplied by the manufacturer and fitted using a non-linear least-squares method to a model describing one set of binding sites. Stopped-flow kinetics Stopped-flow measurement were obtained using a TgK Scientific stopped-flow system (model SF-61DX2). Ac-AChBP was excited at 280 nm, and emission was recorded with a band filters WG320 and VG11. Changes in fluorescence emission intensity were fit to a first- (nicotine) or a second- (VUF9432) order equation. Electrophysiology To probe effects of VUF9432 and AO at the α7 nAChR receptors, experiments were conducted at Xenopus oocytes expressing the homomeric human α7 nAChRs. Expression was obtained by intranuclear injection of 10 nl of a solution containing the cDNA encoding for the human α7 subunit at a concentration of 0.2 μg ml −1 using an automated injector (roboinject, Multichannelsystems, Germany). Oocyte preparation and injection was done using the standard procedures as previously described [60] . Three or more day later, electrophysiological properties of the cells were assessed using an automated electrophysiological setup (HiClamp, Multichannelsystems, Germany). Recordings electrodes were filled with 3 M KCl and oocytes superfused with OR2 medium containing in mM: NaCl 82.5, KCl 2.5, HEPES 5, CaCl 2 .2H 2 O 1.8, MgCl 2 .6H 2 O 1, pH 7.4. Cells were held at −80 mV, and α7 expression was tested responses by a brief exposure to 1 mM acetylcholine. Cells displaying robust currents were subsequently tested for their sensitivity to the compound. Accession codes: Atomic coordinates and structure factors for the reported crystal structure have been deposited in the Protein Data Bank with accession code 4bfq . How to cite this article: Stornaiuolo, M. et al . Assembly of a π–π stack of ligands in the binding site of an acetylcholine-binding protein. Nat. Commun. 4:1875 doi: 10.1038/ncomms2900 (2013).